Modular structure facilitates mosaic evolution of the brain in chimpanzees and humans Different brain components can evolve in a coordinated manner or they can show divergent evolutionary trajectories according to a mosaic pattern of variation. Understanding the relationship between these brain evolutionary patterns, which are not mutually exclusive, can be informed by the examination of intraspecific variation. Our study evaluates patterns of brain anatomical covariation in chimpanzees and humans to infer their influence on brain evolution in the hominin clade. We show that chimpanzee and human brains have a modular structure that may have facilitated mosaic evolution from their last common ancestor. Spatially adjacent regions covary with one another to the strongest degree and separated regions are more independent from each other, which might be related to a predominance of local association connectivity. Despite the undoubted importance of developmental and functional factors in determining brain morphology, we find that these constraints are subordinate to the primary effect of local spatial interactions. Macroevolutionary studies of neuroanatomy tend to show coordinated variation of different brain structures that are related to developmental constraints [1] . Particular selective pressures, however, have been shown to exert effects on specific regions that result in a mosaic-like pattern of evolution, with diverse structures showing divergent evolutionary trajectories [2] , [3] , [4] , [5] . Brain evolutionary changes will tend to be concerted when different structures are highly integrated due to pleiotropy, genetic linkage or epigenetic processes [6] , which can constraint patterns of brain reorganization. Alternatively, mosaic evolution will be more likely when brain regions are relatively independent from one another, thus giving rise to distinct modules. Modular architectures are expected to facilitate evolution because different traits can respond to selection in diverging ways [7] . Although this relative interdependence of brain components has a macroevolutionary result, it also has a microevolutionary origin and thus requires an intraspecific context to be addressed. Cranial and craniofacial integration and modularity have been extensively investigated in studies of human evolutionary anatomy [6] , [8] , [9] , [10] . Most of these studies, however, lack a critical comparison of the extent to which craniofacial variation is influenced by brain variation. Unlike studies of cranial evolution that can include hominin fossil species, because brain tissue does not fossilize, inferences about hominin brain evolution must rely on the comparison of extant species, that is, chimpanzees and humans. Comparative analyses of extant species can help to identify aspects of brain organization that were present before the divergence of the hominin–panin lineages and those that have diverged across panin and hominin evolution, supplementing information that can be gleaned from endocranial evolution [11] , [12] , [13] , [14] , [15] , [16] , [17] . The field of neuroscience has tended to analyse patterns of covariation, which are relevant to the study of brain networks, from a different perspective and using a different set of methodological tools [18] than those used in anthropology and evolutionary biology. Elements within the same network are expected to show coordinated variation, whereas different networks are likely to represent different modules. Studies of structural and functional brain networks are common in the neuroimaging literature [19] , [20] but, in many cases, they overlook evolutionary history. In addition, the methodological advance of neuroimaging approaches in which many network analyses are based has progressed more rapidly than the capacity to infer biologically relevant patterns from these techniques [21] . For this reason, it is especially important to study brain variation in the context of general evolutionary theory, using the same theoretical framework and methodological tools employed in the analysis of other structures and organisms. Geometric morphometric techniques provide a suitable methodological framework to evaluate these questions by combining some of the strengths of evolutionary biology and neuroscience approaches. These methods offer a suitable way to evaluate correlated variation among brain regions and provide a different perspective than that offered by scaling analyses of the size of neural structures [1] , [2] , [3] , [4] , [5] . Geometric morphometric methods allow for a multivariate assessment of covariance structure in which the spatial relationships between anatomically homologous locations are maintained across the different steps of the analysis [22] . In this way, not only the size of the different structures defined by homologous landmarks can be incorporated into the analysis of covariation but also their position and orientation within the whole brain and with respect to each other. This allows for a much more complete analysis of covariation patterns, as, once overall size-related modifications are accounted for, different structures can show correlated variation that is not directly reflected in size increases or decreases. In this study, we used a three-dimensional (3D) geometric morphometric framework to analyse and compare intraspecific patterns of covariation between brain regions based on in vivo magnetic resonance imaging (MRI) scans of chimpanzee and human brains. We used both a hypothesis-free and a hypothesis-based approach, in which we compared three competing models based on different biological assumptions regarding the factors driving anatomical covariation: evolutionary and developmental factors, structural factors or functional factors. Our results show that chimpanzee and human brains are characterized by a very weak level of integration. The structural model is the only one that shows significant modularity and, within this model, correlated variation is especially low between spatially separated regions. The observed modular organization, which is based predominantly on spatial proximity, may allow for relatively independent variation of non-adjacent regions, thus facilitating mosaic evolution. We suggest this architecture to have permitted the sequential acquisition along hominin evolution of traits that are typical of modern human brains. Hypothesis-free assessment of integration The distribution of variance across the different principal components (PCs) of shape variables corresponding to all landmarks ( Fig. 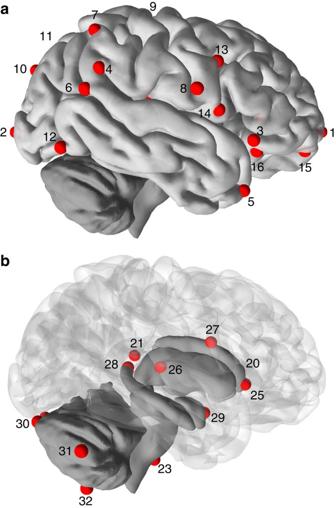Figure 1: Landmarks used in this study. Cortical (a) and subcortical landmarks (b) are represented on a human brain. Landmarks 17, 18 and 19 (insular landmarks), and 22 and 24 are not represented. Note that the definition of landmarks 10, 11, 15 and 16 is not exactly the same in chimpanzees and humans. 1 , Table 1 ) was used to obtain a general assessment of the degree of integration of chimpanzee and human brains before evaluating biological models of modularity ( Fig. 2 , Supplementary Table 1 ). This distribution demonstrates that no single PC accounts for a substantial proportion of variance in the samples ( Fig. 3 ). On the contrary, different PCs account for low and similar proportions of variance both for chimpanzees and humans, with the first PC accounting for no more than 15% of variance. This points to a weakly integrated structure overall in both species. Figure 1: Landmarks used in this study. Cortical ( a ) and subcortical landmarks ( b ) are represented on a human brain. Landmarks 17, 18 and 19 (insular landmarks), and 22 and 24 are not represented. Note that the definition of landmarks 10, 11, 15 and 16 is not exactly the same in chimpanzees and humans. Full size image Table 1 Definition of anatomical landmarks. 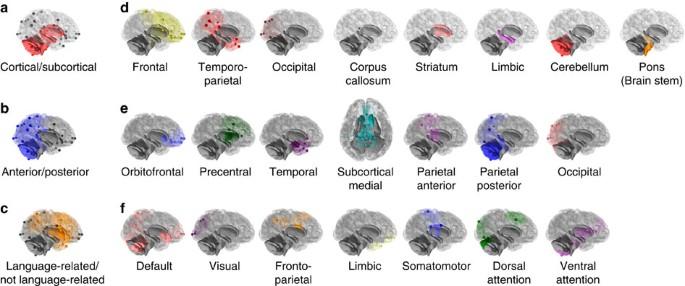Figure 2: Modularity models. (a) Large-scale EvoDevo model; (b) large-scale structural model; (c) large-scale functional model; (d) fine-scale EvoDevo model; (e) fine-scale structural model; (f) fine-scale functional model. Similarly coloured modules are not equivalent across the three models. Note that the limbic module is not equivalent in the EvoDevo model and in the functional model. Note as well that our parcellation in the fine-scale functional model does not match exactly those in refs25,62and63because our parcellation uses an interpolation based on the anatomical landmarks that are represented in each network. Full size table Figure 2: Modularity models. ( a ) Large-scale EvoDevo model; ( b ) large-scale structural model; ( c ) large-scale functional model; ( d ) fine-scale EvoDevo model; ( e ) fine-scale structural model; ( f ) fine-scale functional model. Similarly coloured modules are not equivalent across the three models. Note that the limbic module is not equivalent in the EvoDevo model and in the functional model. Note as well that our parcellation in the fine-scale functional model does not match exactly those in refs 25 , 62 and 63 because our parcellation uses an interpolation based on the anatomical landmarks that are represented in each network. 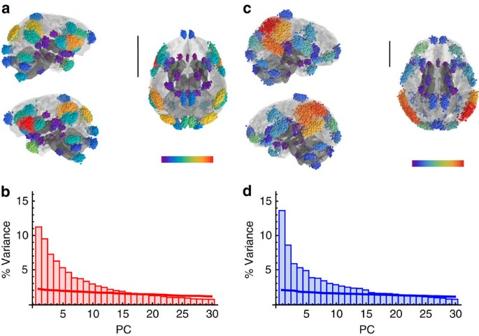Figure 3: Hypothesis-free evaluation of integration. (a) Procrustes-superimposed landmarks corresponding to the chimpanzee sample (n=189) before symmetrizing configurations of landmarks; (b) scree plot showing the percentage of variance (% Variance) explained by each PC in the chimpanzee sample (red); (c) Procrustes superimposed landmarks corresponding to the human sample (n=189) before symmetrizing configurations of landmarks; (d) scree plot showing the distribution of variance across different PCs in the human sample (blue). Ina,clandmarks have been Procrustes-superimposed and later translated to the original space of the individual represented as a brain surface model. Scale bars, 5 cm. Landmarks are colour-coded to represent dispersion around their location in the mean or consensus shape of each sample (red represents high values and purple represents low values). This dispersion is highest at the inferior extreme of the left precentral sulcus in chimpanzees and at the most posterior and superior extreme of the right superior temporal sulcus in humans. Inb,dsolid lines represent the scree plots obtained from a random model of variation. Only the first 30 PCs are represented. Full size image Figure 3: Hypothesis-free evaluation of integration. ( a ) Procrustes-superimposed landmarks corresponding to the chimpanzee sample ( n =189) before symmetrizing configurations of landmarks; ( b ) scree plot showing the percentage of variance (% Variance) explained by each PC in the chimpanzee sample (red); ( c ) Procrustes superimposed landmarks corresponding to the human sample ( n =189) before symmetrizing configurations of landmarks; ( d ) scree plot showing the distribution of variance across different PCs in the human sample (blue). In a , c landmarks have been Procrustes-superimposed and later translated to the original space of the individual represented as a brain surface model. Scale bars, 5 cm. Landmarks are colour-coded to represent dispersion around their location in the mean or consensus shape of each sample (red represents high values and purple represents low values). This dispersion is highest at the inferior extreme of the left precentral sulcus in chimpanzees and at the most posterior and superior extreme of the right superior temporal sulcus in humans. In b , d solid lines represent the scree plots obtained from a random model of variation. Only the first 30 PCs are represented. Full size image The difference between the proportion of variance explained by the first and second PCs is slightly higher in humans than in chimpanzees, thus pointing to a slightly higher degree of integration in humans. These differences, however, are moderate between both species, as revealed by covariance matrix correlations between chimpanzees and humans of 0.68 (matrix permutation test with landmark permutation: P <0.001, which leads to a rejection of the null hypothesis of total dissimilarity). This value demonstrates that covariance matrices are significantly similar in both species. Theoretical and comparative neuroanatomical studies suggest that allometric effects of increased brain size may lead to a higher degree of modularity in the neocortex of large brains, since communication is more efficient across small areas of the cortex than between distant areas [23] . In this context, it is notable that human brains show a slightly higher level of integration than chimpanzees. Although it is tempting to speculate about a more distributed organization of brain networks in humans, differences between chimpanzees and humans implied in these results are minor and it is not clear that the distribution of variance we observe for the whole brain in this analysis can be interpreted to reflect the organization of functional networks, as it is described in the following section. Evaluation of modularity and comparison between models Given the previous results indicating weak integration in chimpanzee and human brains, which is a necessary but not sufficient prerequisite for a modular structure, we evaluated three competing models of modularity that are based on different biological assumptions concerning the causes of anatomical parcellation ( Fig. 2 , Supplementary Table 1 ). Each of these models was evaluated at a large scale (that is, using only two different modules) and at a fine scale (that is, using a larger number of modules corresponding to fine-grained systems). (1) An EvoDevo model evaluated covariation between brain structures with different developmental origins and evolutionary trajectories. (2) A structural model analysed modularity based on spatial proximity under the assumption that anatomically adjacent regions covary to a stronger degree than regions separated by long distances. (3) A functional model evaluated modularity among different functional areas under the assumption that anatomical variation might reflect underlying functional connectivity. This model evaluated covariation between regions functionally involved in language processing and production in humans and regions without that functional involvement [24] (large-scale model), or between modules that were defined based on resting-state functional connectivity [25] (fine-scale model). Only the structural model showed significantly higher modularity than random partitions of the sample for chimpanzees and humans, and for the large-scale and fine-scale models ( Fig. 4 , Table 2 ). Several studies have demonstrated that modularity is usually influenced by developmental origin [26] , which, in this case, corresponds to embryological segmentation of brain regions. In our analyses, evolutionary and developmental factors, however, seem to play a minor role in driving patterns of covariation within each species when compared with spatial proximity ( Table 2 ). Similarly, functional networks do not show a major role in determining patterns of correlated variation in comparison with structural factors. Most cerebral shape changes evaluated in our study describe variation in the relative position of sulci and gyri that, in the end, are related to the expansion or reduction of certain regions. A few studies have tried to connect brain macro- and microstructure in humans [27] , [28] , chimpanzees [29] and other primates [30] , but more conclusive associations await larger sample sizes and a multivariate approach to understand intraspecific variation. Sulcal variation has been demonstrated to be a reasonable predictor of cytoarchitecture for primary and secondary regions such as visual, somatosensory and motor areas [28] ; however, it appears to be less reliable to identify higher order cognitive areas in both chimpanzees and humans [28] , [31] . In any case, sulcal and gyral variation is likely to have an indirect relevance as a macromorphological manifestation of functionally key microstructural changes. 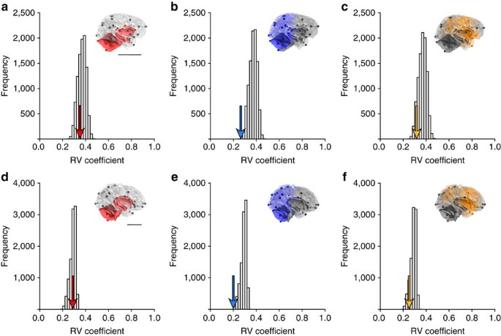Figure 4: Hypothesis-based evaluation of modularity in the large-scale models. (a) EvoDevo model in chimpanzees; (b) structural model in chimpanzees; (c) functional model in chimpanzees; (d) EvoDevo model in humans; (e) structural model in humans; (f) functional model in humans. Fora–f, arrows represent the actual RV coefficient obtained for the corresponding model, and histograms represent the distribution of RV coefficients yielded by random partitions of landmarks from which thePvalues discussed in the comparison of the models are calculated. Scale bars, 5 cm. Figure 4: Hypothesis-based evaluation of modularity in the large-scale models. ( a ) EvoDevo model in chimpanzees; ( b ) structural model in chimpanzees; ( c ) functional model in chimpanzees; ( d ) EvoDevo model in humans; ( e ) structural model in humans; ( f ) functional model in humans. For a – f , arrows represent the actual RV coefficient obtained for the corresponding model, and histograms represent the distribution of RV coefficients yielded by random partitions of landmarks from which the P values discussed in the comparison of the models are calculated. Scale bars, 5 cm. Full size image Table 2 RV coefficients and P values (based on permutation tests) obtained for the three modularity models at a large and fine scale. Full size table Among the large-scale structural models that we tested, only a model separating anterior from posterior landmarks shows significant modularity for both species ( Table 3 ). Models separating medial from lateral landmarks, and superior from inferior landmarks, do not show significant levels of modularity. A spatial distance-based model of modularity is a default expectation for most biological systems [32] ; however, anterior–posterior partitions of landmarks show much clearer parcellation than other partitions ( Table 3 ). Other features of anatomical variation have been demonstrated to show a rostrocaudal gradient in primate (including human) brains [33] , a morphological continuum that is likely related to gene expression gradients [34] . Similarly, numbers of neurons in the neocortex show a rostrocaudal gradient in humans [27] and nonhuman primates [35] . This rostrocaudal partition is partially related to developmental factors such as the timing of neurogenesis, as demonstrated by the separation in our EvoDevo model of a frontal, temporoparietal and occipital regions, a parcellation that is consistent with evolutionary and developmental regionalization of the neocortex [36] . However, more local factors appear to drive anatomical covariation, as the EvoDevo model does not show significant modularity in either species. Table 3 RV coefficients and P values (based on permutation tests) obtained for different structural divisions of landmarks. Full size table Organization of structural modules When covariation between the different modules demarcated in the fine-scale structural model is evaluated through pairwise comparisons, it can be observed that modules are not completely independent from each other in spite of the significant degree of modularity observed for this partition of landmarks ( Supplementary Tables 2 and 3 ). On the contrary, all the modules covary significantly with each other with a strength that is influenced by spatial proximity. This is represented in graphical models, where significant edges with high bootstrap support are mostly those grouping spatially adjacent modules ( Fig. 5 ). Graphical models show the separation of anterior versus posterior areas in both the species. In humans, the anterior and posterior parts of the brain are more clearly regionalized than in chimpanzees. The anterior complex in humans includes the orbitofrontal and precentral modules, and the posterior one includes both parietal modules. In chimpanzees, the posterior complex appears to be more clearly spatially defined than the anterior one. The posterior complex includes the occipital and superior parietal modules, whereas the anterior complex includes both frontal modules but also the subcortical medial and inferior parietal modules. These association patterns might indicate an inverse relationship between distance and strength of covariation. However, although this trend exists in both species, it is not significant ( Supplementary Fig. 1 ). 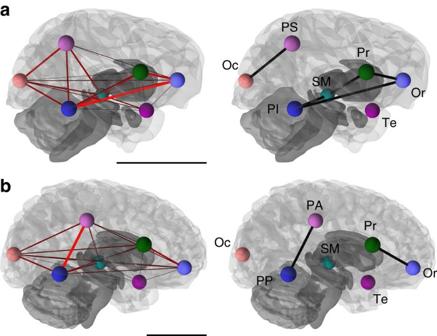Figure 5: Graphical models showing pairwise correlations between structural modules. (a) Chimpanzees; (b) humans. Ina,bthe model to the left shows pairwise RV coefficients between all modules, with edge thicknesses and colour intensity proportional to pairwise RV values (red thick edges represent the highest RV values). Models to the right include only edges showing significant partial correlations between structural modules. Graphical models are superimposed on 3D models of chimpanzee and human brains. Coloured spheres represent the centroid of each structural module (Or: orbitofrontal; Pr: precentral; Te: temporal; SM: subcortical medial; PS: parietal superior; PI: parietal inferior; PA: parietal anterior; PP: parietal posterior; Oc: occipital). (a) Chimpanzees: two complexes are identified, a posterior one including the superior parietal and occipital modules, and an anterior complex that includes frontal modules, as well as subcortical medial and inferior parietal modules. (b) Humans: two complexes are identified, an anterior one formed by both frontal modules and a posterior one formed by both parietal modules. Scale bars, 5 cm. Figure 5: Graphical models showing pairwise correlations between structural modules. ( a ) Chimpanzees; ( b ) humans. In a , b the model to the left shows pairwise RV coefficients between all modules, with edge thicknesses and colour intensity proportional to pairwise RV values (red thick edges represent the highest RV values). Models to the right include only edges showing significant partial correlations between structural modules. Graphical models are superimposed on 3D models of chimpanzee and human brains. Coloured spheres represent the centroid of each structural module (Or: orbitofrontal; Pr: precentral; Te: temporal; SM: subcortical medial; PS: parietal superior; PI: parietal inferior; PA: parietal anterior; PP: parietal posterior; Oc: occipital). ( a ) Chimpanzees: two complexes are identified, a posterior one including the superior parietal and occipital modules, and an anterior complex that includes frontal modules, as well as subcortical medial and inferior parietal modules. ( b ) Humans: two complexes are identified, an anterior one formed by both frontal modules and a posterior one formed by both parietal modules. Scale bars, 5 cm. Full size image It is important to note that our results are based only on patterns of correlated variation in the position of the anatomically homologous landmarks that we have examined. However, potential concerns about different scaling methods of other commonly evaluated variables (such as volumetric measures), which can have a strong impact on results, are taken into account in our geometric morphometric approach, as landmark configurations (and, hence, brain morphologies represented by them) are scaled at the initial steps of the analysis. In fact, our results have some similarities with the ones obtained when using variables that are more typically evaluated in neuroscience, such as regional volume, surface area or cortical thickness ( Supplementary Methods and Supplementary Table 4 ). It has to be noted, nonetheless, that results based on these different variables are not expected to match because they have different genetic, developmental and evolutionary underpinnings [37] . As the landmark-based model, the volume-, area- and thickness-based models show a predominance of significant edges between modules that are physically adjacent ( Fig. 5 and Supplementary Fig. 2 ). The volume-based model shows the clearest similarity to the landmark-based model, especially in the low number of significant partial correlations and in the separation of an anterior and a more posterior complex. Surface area- and cortical thickness-based models, however, do not show a clear parcellation of anterior and posterior regions. Intraspecific analyses of correlated variation provide a fundamental way to evaluate the problem of concerted versus mosaic evolution of the brain because macroevolutionary patterns of covariation are grounded in the variation that is observed within species. Intraspecific studies can help to elucidate whether different regions of the brain are more or less prone to evolve in a coordinated or independent way. Our observation of modular variation in chimpanzee and human brains is in line with reports of independent variation and regulation between brain components based on quantitative genetic analyses of mice [38] . Our results, however, shift the focus from relative independence of developmentally distinct regions to relative independence of spatially separated regions. This proximity-dependent modular organization might be a particularity of great ape and human brains because of their large size and high morphological complexity as compared with other mammalian brains. The spatial relationships among ontogenetically related structures, which would be initially expected to show the highest relative independence, ultimately become altered because of the high morphological and connectional complexity of the large and gyrified brains of chimpanzees and humans. For example, prefrontal and occipital regions of the cerebral cortex are spatially separated along the rostrocaudal axis, even though they share a common developmental origin from the dorsal telencephalon. Our results show that the frontal cortical region covaries most with other frontal regions, and that the occipital neocortical areas covary with the posterior region of the cerebellum, which is derived from the rhombencephalon, in spite of their different developmental and evolutionary trajectories. A similar lack of cortical-subcortical independent modularity has been described using a similar methodological approach in midsagital sections of human brains, where a model of spatially contiguous parietal landmarks has been suggested to show the highest independence from the rest of the brain [39] . These results highlight the important influence of basic local spatial interactions in constraining brain morphological variation. These interactions can include biophysical properties of axonal connections, which are likely to cause correlated changes in the areas that they connect [40] , regardless of whether they are corticocortical or corticosubcortical connections. Landmarks included within each structural module in our study are mostly those located on adjacent sulci and gyri. Therefore, the observation of proximity-dependent modularity might be related to the presence of short association fibres (also called U-fibres) between neighbouring cortical areas, which have been proposed to be increased in human brains [41] . It has to be noted that similar (and probably homologous) U-fibres have been described in the rhesus macaque, and that these fibres are probably highly conserved during primate brain evolution [42] , thus leading to the similar patterns of covariation observed in chimpanzees and humans. The structural model of modularity, however, includes within certain modules regions of the brain outside of the neocortex that are not connected by short association fibres. A potential factor causing correlated variation between adjacent regions not connected by U-fibres and even with different developmental origins is spatial packing, which can have a role in causing covariation between neighbouring regions of the occipital cortex and the cerebellum. In this regard, our definition of spatial packing is slightly more general than the classically studied relationship between basicranial flexion and encephalization [43] , and it makes reference to the physical constraints imposed by the limited available space within the braincase on large brains. Network analyses of the human skull have shown the importance of spatial relationships and proximity to account for the modular structure of correlated shape changes [44] . These and our results, however, contrast with the pattern of pervasive genetic integration described for human skulls, which has been proposed to drive the evolution of cranial shape [10] . Owing to the reciprocal interaction between cerebral and cranial development [45] , related patterns of covariation can be expected between the brain and the skull. One possible explanation for this apparent difference is that our analyses of pairwise comparisons actually do demonstrate that all modules covary significantly with each other ( Supplementary Tables 2 and 3 ). Nonetheless, the strength of this covariation differs across different modules, with the highest values corresponding to spatially adjacent regions and the lowest values to distant regions ( Fig. 5 ). These results are supportive of spatially distant brain areas varying more independently from each other than adjacent areas but not of completely independent variation. In addition, the relationship between genetic and phenotypic integration is not entirely clear [46] . It has been previously demonstrated that fluctuating asymmetry, which can be indicative of developmental plasticity and a proxy for non-genetic variation, accounts for a substantial proportion of morphological variance in chimpanzee and, even more so, in human brains [47] . In this light, it is important to note that the human cortical surface shows a clear distance-dependent hierarchical organization when genetic correlations are studied but a less clear structure based on phenotypic correlations [48] . One of the main differences reported between phenotypic and genetic correlations is allocated at the posterior perisylvian area, where a very asymmetric pattern is observed in humans for phenotypic correlations but not for genetic correlations [48] . This observation is consistent with previous reports of increased fluctuating asymmetry of postsylvian regions in humans [47] . Environmental effects are known to modify the phenotype of brain morphology, which is initiated by genetic interactions. Non-genetic influences can give rise to a more modular pattern of variation than expected solely on the basis of genetics. If the adult brain phenotype is affected by environmental interactions, which are heavily dependent on social and cultural influences in humans, it is possible that different brain regions respond in a relatively independent way to non-genetic factors, thus giving rise to the observed modular pattern of phenotypic variation. One of the most consistent results in our study is the general similarity in brain modular structure between chimpanzees and humans ( Figs 3 , 4 , 5 ; Tables 2 and 3 ), a result that strikingly contrasts with reported differences in craniofacial integration [49] . Similar patterns of brain modularity are especially relevant because anatomical differences in chimpanzee and human brains are clear [47] , [50] ; however, they seem to be built upon fundamental symplesiomorphic structural interactions that were probably present in the hominin–panin last common ancestor. The predominance of modularity based on spatial proximity may permit evolutionary flexibility, allowing for anatomical and functional differences that have arisen between chimpanzee and human brains. Studies of the mammalian skull have demonstrated that Homo and Pan show the lowest levels of integration and constraints and the highest levels of evolutionary flexibility not only across primates but also across most mammals [51] , a result that is compatible with our results showing a modular architecture in chimpanzee and human brains. This modular organization might allow for increased responsiveness of the brain to particular selective pressures [51] , facilitating mosaic evolution. Mosaic variation is indeed observed in the hominin fossil record through the sequential appearance of traits considered to be typical of modern human brains. A reorganization of the occipital areas, represented in fossil endocasts as a change in the position of the lunate sulcus marking a reduction of the primary visual cortex, can be one of the first acquisitions during hominin brain evolution, perhaps already present in Australopithecus afarensis and A. africanus [11] (but see ref. 14 ). Significant orbitofrontal reorganization has been suggested to be present in A. sediba [52] and is likely to have occurred during the transition between Australopithecus and early Homo [13] . Both occipital and orbitofrontal reorganizations are observed in the hominin fossil record before a substantial increase in brain size (and a likely related increase in gyrification) is observed in H. erectus . Both Neanderthals and modern humans show substantial frontal broadening [53] ; therefore, it can be parsimoniously assumed that this trait originated before the divergence of both species. An anterior projection of the temporal poles [9] , and a general globularization of the brain, which involves both a frontal bulging and a parietal reorganization [16] , [17] , [54] , have been proposed to be recent acquisitions in human evolution, only observed in H. sapiens . Other traits that are not visible in endocasts are likely to have evolved as well in a sequential, mosaic manner, facilitated by the absence of a general, large-scale strong integration. Our results provide an explanation through which the interspecific patterns of variation observed in the hominin fossil record can be explained on the basis of intraspecific variation in brain anatomy. Material A sample of 189 chimpanzees ( Pan troglodytes; 117 females, 72 males; age rage 6–53 years old) and 189 humans ( H. sapiens; 113 females, 76 males; age range 18–60 years old) was studied through in vivo MRI scans. The number of human subjects was chosen to match the number of available chimpanzee scans. Chimpanzees housed at the Yerkes National Primate Research Center (YNPRC) in Atlanta, GE, and at the University of Texas MD Anderson Cancer Center (UTMDACC) in Bastrop, TX, were scanned using a 3T scanner (Siemens Trio, Siemens Medical Solutions, Malvern, USA) or a 1.5T scanner (Phillips, Model 51, Philips Medical Systems, N.A., Bothell, Washington, USA). Scanning procedures in chimpanzees were approved by the Institutional Animal Care and Use Committees at YNPRC and UTMDACC, and also followed the guidelines of the Institute of Medicine on the use of chimpanzees in research. Chimpanzees showed a variety of hand preferences for different tasks. Human scans were obtained from the OASIS database [55] , selecting only healthy (nondemented) and moderately aged individuals (always younger than 60 years old). All the scans stored in this database belong to right-handed individuals and were acquired with a 1.5T Vision scanner (Siemens, Erlangen, Germany). Informed consent for all participants was obtained in accordance with the guidelines of the Washington University Human Studies Committee in the context of the OASIS project. Technical details of human MRI acquisition, as well as population information, is provided in ref. 55 , whereas the equivalent information for chimpanzee MRI scans is provided in ref. 56 . Geometric morphometrics and modularity models 3D surface models of brain hemispheres for both species were reconstructed using the BrainVISA software [57] . Our analyses were based on a set of 19 bilateral cortical landmarks and 13 subcortical landmarks (5 unilateral and 8 bilateral) defined after refs 47 and 50 ( Fig. 1 , Table 1 ). Although landmark-based geometric morphometric techniques are commonly used in evolutionary and palaeontological studies (and, therefore, in the analysis of skeletal remains), these techniques are readily usable in soft tissues, such as brains, as long as homologous locations can be defined and identified. This is the case for the set of landmarks used in our study, which were defined using major sulci in the cortical surface and clearly defined anatomical subdivisions. Cortical landmarks were digitized on 3D reconstructions of the brain surface using IDAV Landmark Editor [58] , whereas subcortical landmarks were digitized on triplanar views of the MRI scans using MIPAV software [59] . Cortical and subcortical landmarks were later merged so as to obtain one single landmark configuration for each individual. Non-shape information corresponding to position, size and orientation was removed using a Procrustes superimposition [60] . Unlike other neuroimaging approaches, no further registration was performed in order to retain all shape variance in the sample, which is the focus of our study. Landmark configurations were symmetrized by averaging the original and mirrored configurations of landmarks for each brain ( Supplementary Data 1 ). Principal components analyses of superimposed Procrustes coordinates were used for a preliminary hypothesis-free assessment of the degree of integration in our samples. Highly integrated structures are characterized by one leading PC explaining most variance in the sample, whereas non-integrated structures show a regular distribution of variance across different PCs [61] . We evaluated modular variation via three competing models based on different biological assumptions ( Fig. 2 , Supplementary Table 1 ), evaluated at a large scale (that is, including only two modules) and at a fine scale (that is, including a larger number of modules). (1) An EvoDevo model evaluated covariation between brain structures with different developmental origins and evolutionary trajectories. In the large-scale case, this model evaluated covariation between cortical and subcortical landmarks. In the fine-scale case, this model evaluated covariation between eight different modules: frontal (cortical), temporoparietal (cortical), occipital (cortical), corpus callosum, striatum, limbic system, pons and cerebellum. The parcellation of cortical landmarks into three different modules (frontal, temporoparietal and occipital) is mainly based on their different evolutionary trajectories. (2) A structural model studied modularity based on spatial proximity. In the large-scale case, this model quantified covariation between rostral and caudal sets of landmarks (corresponding roughly to landmarks located anteriorly or posteriorly to the central sulcus, Fig. 2 and Supplementary Table 1 ). Alternative structural models separating medial from lateral, and superior from inferior, partitions of landmarks were also evaluated. In the fine-scale case, this model included seven modules defined using spatial proximity: orbitofrontal, precentral, temporal, subcortical medial, two parietal modules and occipital. Parietal landmarks were separated into an anterior module and a posterior module in humans, and into a superior module and an inferior module in chimpanzees because of the different spatial relationships among landmarks in both species. (3) A functional model evaluated modularity among areas with different functional involvements. In the large-scale case, this model evaluated covariation between regions involved in language processing and production versus the remaining brain regions. Regions within the language network were selected as those showing positron emission tomography (PET) or functional MRI (fMRI) activation for specific language-related tasks [24] . In the fine-scale case, modules were defined using models of cortical parcellation based on functional connectivity [25] . This parcellation has been also mapped onto the cerebellum [62] and the striatum [63] . Landmarks in other locations (corpus callosum, pons, hippocampus and amygdala) were not included in this model. In order to design this model of modularity, each landmark was assigned to the functional network to which that anatomical location belonged in the initial parcellation of the cortex [25] , striatum [63] and cerebellum [62] , although extensive variability in the anatomical location of these functional networks has been described [64] . Functional models were defined using information based on humans because equivalent information about functional parcellation in the chimpanzee brain is not available, although some studies of intrinsic connectivity networks have revealed striking similarities between humans, chimpanzees, baboons and capuchins [65] . Nonetheless, this human-based definition of the model may be involved in the higher level of modularity observed for humans in the fine-scale functional model. A similar result might be expected for the large-scale functional model, which is based on the definition of language-related areas in humans [24] ; however, in that case, both chimpanzees and humans show similar, marginally significant results. Quantification of integration and modularity Correlated variation between modules was evaluated using the RV coefficient [66] . This approach measures the strength of correlated changes in the position of landmarks regardless of the direction of those changes. The RV coefficient is described as a multivariate analogue to the squared correlation coefficient, for which a value of 0 indicates complete modularity and a value of 1 indicates complete integration. These extreme values, however, are orientative, and the significance of the evaluated patterns of modularity was assessed using permutation tests. P values for modularity models were calculated as the proportion of 10,000 random partitions of landmarks (which observe bilateral symmetry) showing higher modularity (lower RV value) than the evaluated model. For models including more than two modules, a multiset RV coefficient was used [66] . Because size, age and sex have a quantitatively very minor effect on the evaluated morphologies [47] ( Supplementary Tables 5 and 6 ), we did not correct shape variables for allometry, age or sex. Similarly, significant, although quantitatively very minor, differences located mainly at occipital landmarks were observed between chimpanzee brains scanned with a 1.5T versus a 3T scanner. These differences have a quantitative value of less than half of the smallest interindividual Procrustes distance observed in the sample ( Supplementary Table 6 ). Even though these differences appear to be minor, we repeated our analyses within each of the samples to confirm that no scan-related bias influences our results. These additional analyses showed that modularity patterns observed in chimpanzees are consistent regardless of the type of scanner ( Supplementary Table 7 ). Models showing significant modularity are not necessarily formed by modules that are completely independent from each other. Therefore, RV coefficients between each pair of modules were calculated for the structural model. Significance was evaluated using permutation tests for the null hypothesis of complete independence between modules. Pairwise RV coefficients were calculated using a common Procrustes superimposition for all the modules. The geometry of those patterns of covariation was graphically depicted using a graphical modelling approach, which has been extensively used in the study of brain networks [19] . Graphical models were obtained with a modification of the approach presented in ref. 67 based on between-module pairwise RV coefficients. These coefficients were used to calculate partial correlations, which measure the correlation of two variables conditioned on all other variables, and their significance was assessed using the edge exclusion deviance criterion [67] . Consensus graphical models were obtained to account for the variability in estimating RV coefficients. Only edges showing significant partial correlations ( P <0.05) in more than 90% of 1,000 bootstrap resamplings of the original chimpanzee and human populations were represented. Analyses were performed in MorphoJ [68] and in Mathematica using the Geometric Morphometrics package written by P.D. Polly [69] and the Modularity package written by P.D. Polly and A. Goswami [70] . How to cite this article: Gómez-Robles, A. et al . Modular structure facilitates mosaic evolution of the brain in chimpanzees and humans. Nat. Commun. 5:4469 doi: 10.1038/ncomms5469 (2014).